The lncRNAMIR31HGregulates p16INK4Aexpression to modulate senescence Oncogene-induced senescence (OIS) can occur in response to oncogenic insults and is considered an important tumour suppressor mechanism. Here we identify the lncRNA MIR31HG as upregulated in OIS and find that knockdown of MIR31HG promotes a strong p16 INK4A -dependent senescence phenotype. Under normal conditions, MIR31HG is found in both nucleus and cytoplasm, but following B-RAF expression MIR31HG is located mainly in the cytoplasm. We show that MIR31HG interacts with both INK4A and MIR31HG genomic regions and with Polycomb group (PcG) proteins, and that MIR31HG is required for PcG-mediated repression of the INK4A locus. We further identify a functional enhancer, located between MIR31HG and INK4A , which becomes activated during OIS and interacts with the MIR31HG promoter. Data from melanoma patients show a negative correlation between MIR31HG and p16 INK4A expression levels, suggesting a role for this transcript in cancer. Hence, our data provide a new lncRNA-mediated regulatory mechanism for the tumour suppressor p16 INK4A . The mammalian genome encodes thousands of long non-coding RNAs (lncRNAs), which are transcribed and processed in a manner similar to messenger RNAs, but lack the protein-coding potential. Some of these transcripts are essential factors for the regulation of important cellular processes such as proliferation, differentiation or development, as well as a broad range of diseases including cancer [1] , [2] , [3] . LncRNAs participate in a broad spectrum of gene-regulatory functions such as epigenetic activities, translational regulation or scaffolding/decoy functions [4] , [5] , [6] . As transcriptional regulators, a number of lncRNAs regulate the transcription of neighbouring genes by cis -acting mechanisms [7] , [8] , [9] , but may also act in trans without affecting neighbouring genes [10] , [11] , [12] , [13] . Cellular senescence is a state of irreversible growth arrest [14] , which can be triggered by different stimuli, such as telomere shortening, DNA damage, oxidative stress or oncogene activation [15] . In addition, senescence has recently been demonstrated to have a role in tissue patterning and remodelling during normal development [16] , [17] . Oncogene-induced senescence (OIS) was first reported by Serrano et al. [18] when they observed primary human and mouse fibroblasts undergoing senescence following expression of an oncogenic form of RAS. Later reports showed that many other oncogenes might cause OIS both in vitro and in vivo [19] , [20] . OIS is considered a barrier against tumorigenesis. In support of this, senescent cells are present in pre-malignant tissues and not in tumour cells, indicating that senescence must be bypassed by additional tumorigenic alterations to progress towards malignancy [19] , [20] . Senescent cells have been found to secrete interleukins, metalloproteases and other cytokines as part of the senescence-associated secretory phenotype (SASP) and these factors are known to stimulate cancer progression in a non-cell autonomous manner [15] , [21] , [22] . Therefore, senescence may either fuel or halt tumour progression and this may depend on the age of the organism [23] , [24] . Cellular senescence is primarily dependent on two tumour suppressor pathways: p14 ARF /p53 and p16 INK4A /pRB, both of which mediate cell cycle arrest. The upstream proteins of both pathways, p16 INK4A and p14 ARF , together with an additional tumour suppressor protein p15 INK4b , are encoded by the same locus INK4B-ARF-INK4A at human chromosome 9p.21. This locus is tightly regulated by the Polycomb group proteins (PcGs) [25] , [26] , [27] , which are responsible for its transcriptional repression in normal cells. During senescence, the Polycomb repressive complexes 1 and 2 (PRC1 and PRC2) are dissociated from the chromatin, resulting in transcriptional activation [26] . Notably, the lncRNA ANRIL (antisense non-coding RNA in the INK4 locus) is encoded in antisense orientation by the same locus [28] and affects the epigenetic silencing of p15 INK4b (ref. 29 ). ANRIL has been demonstrated to mediate the recruitment of chromatin silencing machinery to the INK4 locus and to suppress the expression of p15 INK4B (refs 29 , 30 ); however, its role during senescence remains unclear. Recently, the lncRNA UCA1 has been reported to interact with hnRNPA1 and to increase p16 INK4A mRNA stability by preventing its degradation [31] . In another recent report, PANDA lncRNA has been shown to regulate senescence entry and exit, and to interact with the scaffold-attachment factor A [32] . Other lncRNAs have been identified to be involved in cellular senescence, although their mechanisms of action remain uncharacterized [33] . The importance of the INK4/ARF locus and the interplay between OIS and cancer prompted us to further investigate lncRNAs deregulated in OIS. We identify a number of deregulated lncRNAs during B-RAF-induced OIS. Among these, MIR31HG / LOC554202 is upregulated in OIS, whereas the knockdown of MIR31HG promotes a p16 INK4A -dependent senescence phenotype. Under normal conditions MIR31HG is located in both the nucleus and the cytoplasm, whereas upon B-RAF expression MIR31HG is almost exclusively localized in the cytoplasm. We demonstrate that the MIR31HG transcript interacts with the genomic regions INK4A and MIR31HG , and with PcG proteins, and that MIR31HG is required for PcG binding and repression of the INK4A locus. We further identify an enhancer, located between MIR31HG and the INK4A loci, which is activated during OIS and directly interacts with the MIR31HG locus. Finally, we found an anti-correlation between MIR31HG and p16 INKA RNA expression in melanoma, suggesting a role for this transcript in cancer. Together, our results provide a new lncRNA-mediated regulatory mechanism for the tumour suppressor p16 INK4A during OIS. Our findings highlight the role of lncRNAs acting as transcriptional regulators in critical processes such as cellular senescence and cancer. MIR31HG is induced during OIS To identify lncRNAs with a role in OIS, we used immortalized human diploid fibroblasts, TIG3-hTERT, expressing a constitutively activated form of the mouse B-RAF (V600E) fused to the oestrogen receptor (ER:B-RAF). Addition of 4-hydroxitamoxifen (4-OHT) activates B-RAF and consequently induces OIS. This senescent phenotype includes activation of the enzyme β-galactosidase, induction of p16 INK4A expression, growth arrest and formation of senescence-associated heterochromatin foci (SAHFs) characterized by high levels of H3K9me3 ( Supplementary Fig. 1a–d ). RNA sequencing in OIS and control cells revealed that 655 protein-coding and 131 non-coding RNAs were affected by B-RAF overexpression (log 2 -fold change >±1.5, false discovery rate <0.05; Fig. 1a and Supplementary Data 1 ). Quantitative reverse transcriptase–PCR (qRT–PCR) validation of a gene set known to be relevant for senescence confirmed the robustness of the model ( Fig. 1b ). The majority of the lncRNAs deregulated in OIS corresponded to long-intergenic RNAs (lincRNAs) and antisense transcripts ( Fig. 1c ). One of the top hits identified was the lincRNA MIR31HG (previously known as LOC554242 (ref. 34 ; Fig. 1d ). Interestingly, this lncRNA is located on chromosome 9 (9p21.3), ∼ 400 kb away from the INK4A locus, which prompted us to investigate it further. We confirmed by qRT–PCR that this transcript was more than eightfold upregulated in OIS ( Fig. 1e ). Using absolute quantification with in-vitro -transcribed MIR31HG as a standard curve for qRT–PCR analyses, we observed that there are ∼ 40 copies of MIR31HG in control cells and 250 in 4-OHT-treated cells ( Fig. 1f ). Further characterization of MIR31HG revealed that it is poly-adenylated ( Supplementary Fig. 1e ) and located both in the cytoplasm and the nucleus ( Fig. 1g ). Using BJ foreskin fibroblast cells from early, intermediate and late passages, we observed an upregulation of MIR31HG during replicative senescence, suggesting that the induction of this lncRNA may be a common feature of different types of senescence ( Supplementary Fig. 1f ). 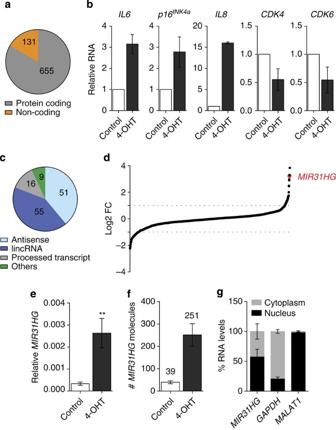Figure 1: The lncRNAMIR31HGis induced during OIS. (a) Pie chart representation of the number of protein-coding and non-coding RNAs deregulated during OIS (log2-fold change >±1.5, false discovery rate (FDR) <0.05). (b) qRT–PCR analysis ofIL-6,p16INK4A,IL-8,CDK4andCDK6in cells treated with 4-OHT relative to cells treated with ethanol as vehicle (control). Data were normalized to housekeeping genes and the levels in control cells set to 1. (c) Diagrammatic representation of the different classes of lncRNAs deregulated during senescence. (d) Representation of all of the lncRNAs altered during OIS with FDR<0.05.MIR31HG(red) was identified as one of the top hits. The dotted lines indicate log2FC=1. (e)MIR31HGRNA levels relative toGAPDHin ethanol- (control) or 4-OHT-treated cells measured by qRT–PCR. (f) The number of molecules ofMIR31HGtranscript in control cells and in 4-OHT-treated cells measured by qRT–PCR using dilutions ofin-vitro-transcribedMIR31HGas standard curve. (g) Percentage of nuclear and cytoplasmic RNA levels ofMIR31HG,GAPDHandMALAT1measured by qRT–PCR after cell fractionation. The graph shows the average of three independent experiments. (b,e–g) The results are from three independent biological experiments and are represented as mean±s.e.m. Student’st-test,**P<0.01. Figure 1: The lncRNA MIR31HG is induced during OIS. ( a ) Pie chart representation of the number of protein-coding and non-coding RNAs deregulated during OIS (log 2 -fold change >±1.5, false discovery rate (FDR) <0.05). ( b ) qRT–PCR analysis of IL-6 , p16 INK4A , IL-8 , CDK4 and CDK6 in cells treated with 4-OHT relative to cells treated with ethanol as vehicle (control). Data were normalized to housekeeping genes and the levels in control cells set to 1. ( c ) Diagrammatic representation of the different classes of lncRNAs deregulated during senescence. ( d ) Representation of all of the lncRNAs altered during OIS with FDR <0.05 . MIR31HG (red) was identified as one of the top hits. The dotted lines indicate log2FC=1. ( e ) MIR31HG RNA levels relative to GAPDH in ethanol- (control) or 4-OHT-treated cells measured by qRT–PCR. ( f ) The number of molecules of MIR31HG transcript in control cells and in 4-OHT-treated cells measured by qRT–PCR using dilutions of in-vitro -transcribed MIR31HG as standard curve. ( g ) Percentage of nuclear and cytoplasmic RNA levels of MIR31HG , GAPDH and MALAT1 measured by qRT–PCR after cell fractionation. The graph shows the average of three independent experiments. ( b , e – g ) The results are from three independent biological experiments and are represented as mean±s.e.m. Student’s t -test, **P< 0.01. Full size image MIR31HG knockdown induces a senescence phenotype To analyse the physiological relevance of this lincRNA in senescence, we knocked down MIR31HG in TIG3-hTERT-ER:B-RAF without 4-OHT treatment, using two independent small interfering RNAs (siRNAs) and assessed a senescence phenotype 72 h post transfection, where we obtained a knockdown efficiency of ∼ 70%–80% ( Fig. 2a ). We observed that knockdown of MIR31HG reduces cell growth in a manner similar to the induction of B-RAF ( Fig. 2b ). This decrease in cell number was not due to apoptosis, as no difference in the percentage of sub-G1 phase cells was detected ( Supplementary Fig. 2a ). Notably, a decrease in the S phase was evident as measured by the diminished incorporation of EdU ( Fig. 2c ). In addition, MIR31HG knockdown cells presented several senescence features including increased β-galactosidase activity ( Fig. 2d ) and significantly increased levels of p16 INK4A expression as detected by immunofluorescence, western blotting and mRNA quantification ( Fig. 2e–g and Supplementary Fig. 2b ). Changes in p14 ARF protein levels were not observed following MIR31HG knockdown ( Supplementary Fig. 2c ). Furthermore, the formation of SAHFs confirmed a strong senescence phenotype in MIR31HG -depleted cells ( Fig. 2h ). Similarly, MIR31HG knockdown in BJ cells led to reduced cell growth and an increase in p16 INK4A protein levels, corroborating our results observed in TIG3 cells ( Supplementary Fig. 2d,e ). 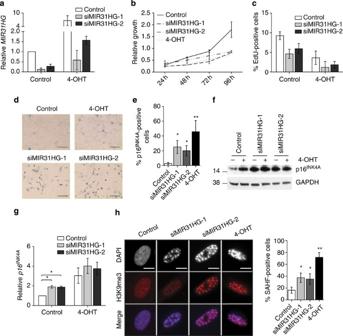Figure 2:MIR31HGknockdown induces a senescence phenotype. (a) RelativeMIR31HGRNA levels in cells transfected with the indicated siRNAs analysed by qRT–PCR in control or 4-OHT-treated cells. Control values were set as 1. Results are represented as mean±s.e.m. from >3 independent experiments. (b) Absorbance levels of crystal violet solution measured at 560 nm from cells transfected with the indicated siRNAs at the designated time points post transfection. (c) Percentage of EdU-positive staining in siRNA-transfected cells with or without 4-OHT treatment. (d) Representative images of the β-galactosidase staining of cells under the indicated conditions 72 h post transfection. Scale bar, 100 μm. (e) Percentage of p16INK4A-positive cells analysed by immunofluorescence 72 h post transfection. (f,g) Western blotting and qRT–PCR analysis of p16INK4Aprotein and mRNA expression, respectively, 72 h post transfection in ethanol or 4-OHT-treated cells. (h) Left, representative images of DAPI (4,6-diamidino-2-phenylindole) and H3K9me3 staining by immunofluorescence in siRNA-transfected cells after 72 h. Right: quantification of the percentage of SAHF-positive cells. At least 150 cells from three independent experiments were counted. Scale bar, 10 μm. All experiments show the mean±s.e.m. from >3 independent experiments. Student’st-test,*P<0.05,**P<0.01. Figure 2: MIR31HG knockdown induces a senescence phenotype. ( a ) Relative MIR31HG RNA levels in cells transfected with the indicated siRNAs analysed by qRT–PCR in control or 4-OHT-treated cells. Control values were set as 1. Results are represented as mean±s.e.m. from >3 independent experiments. ( b ) Absorbance levels of crystal violet solution measured at 560 nm from cells transfected with the indicated siRNAs at the designated time points post transfection. ( c ) Percentage of EdU-positive staining in siRNA-transfected cells with or without 4-OHT treatment. ( d ) Representative images of the β-galactosidase staining of cells under the indicated conditions 72 h post transfection. Scale bar, 100 μm. ( e ) Percentage of p16 INK4A -positive cells analysed by immunofluorescence 72 h post transfection. ( f , g ) Western blotting and qRT–PCR analysis of p16 INK4A protein and mRNA expression, respectively, 72 h post transfection in ethanol or 4-OHT-treated cells. ( h ) Left, representative images of DAPI (4,6-diamidino-2-phenylindole) and H3K9me3 staining by immunofluorescence in siRNA-transfected cells after 72 h. Right: quantification of the percentage of SAHF-positive cells. At least 150 cells from three independent experiments were counted. Scale bar, 10 μm. All experiments show the mean±s.e.m. from >3 independent experiments. Student’s t -test, *P< 0.05, **P< 0.01. Full size image The MIR31HG locus also encodes the microRNA miR-31 in the first intron. The transcription of both the lncRNA and the miRNA is known to be driven by the same promoter [34] . Furthermore miR-31 has previously been reported to be upregulated in OIS [35] . We confirmed that miR-31 expression is increased during OIS but miR-31 expression levels were unaffected by the siRNAs designed against exonic regions of MIR31HG transcript ( Supplementary Fig. 2f ). These results demonstrate that the senescence phenotype induced by the siRNAs is due to MIR31HG knockdown and not due to miR-31 depletion. To address the impact of MIR31HG overexpression in senescence, we created a stable TIG3-B:RAF cell line that overexpressed MIR31HG in a doxycycline-inducible manner. We observed that 72 h doxycycline treatment increases the levels of both nuclear and cytoplasmic MIR31HG in a similar manner ( Supplementary Fig. 3a ). In control proliferating cells, overexpression of MIR31HG did not have an impact on cell proliferation or p16 INK4A protein levels ( Supplementary Fig. 3b , lanes 1–4). However, we observed a diminished p16 INK4A upregulation following 4-OHT treatment ( Supplementary Fig. 3b , lanes 5–8, and Supplementary Fig. 3c ) without affecting cell growth ( Supplementary Fig. 3d ). To investigate whether exogenous MIR31HG could rescue MIR31HG knockdown-induced senescence, we silenced MIR31HG in these cells. The levels of MIR31HG increased approximately fourfold after 72 h doxycycline treatment in cells transfected with control siRNAs ( Supplementary Fig. 3e ). These control cells did not show any evident phenotype measured by p16 INK4A levels and cell proliferation ( Supplementary Fig. 3f–h ). As expected, RNA levels decreased after 72 h knockdown in non-treated cells and were recovered in doxycycline-treated cells for the same period of time ( Supplementary Fig. 3e ). Under these conditions, knockdown of MIR31HG increased p16 INK4A expression at RNA ( Supplementary Fig. 3f ) and protein levels ( Supplementary Fig. 3g ) as previously observed, but not when MIR31HG was simultaneously expressed ( Supplementary Fig. 3f,g ). Moreover, the growth defects observed in knockdown cells after 72 and 96 h transfection were reverted by MIR31HG overexpression ( Supplementary Fig. 3h ). These data demonstrate the specificity of the siRNAs employed against MIR31HG and suggest that cytoplasmatic MIR31HG is not essential for the senescence phenotype. MIR31HG effect in senescence is p16 INK4A dependent To identify the pathways affected by MIR31HG depletion, we performed RNA sequencing from cells transfected with control or MIR31HG siRNAs. From the 83 genes significantly altered by MIR31HG knockdown (log 2 -fold change >±1.5, false discovery rate<0.05), 21 were also affected on B-RAF induction ( Fig. 3a and Supplementary Table 1 ), with only 2 commonly upregulated and 1 commonly downregulated ( Fig. 3b ). We did not find evidence of the induction of broad senescence-related programmes in MIR31HG knockdown cells. In contrast, of the 18 genes oppositely regulated between the two conditions, many encoded cytokines, interleukins and other proteins known to be part of the SASP ( Supplementary Table 2 ) [36] . These were upregulated during OIS but downregulated or unaltered in MIR31HG knockdown cells ( Supplementary Table 2 ). To confirm the absence of SASP in the MIR31HG knockdown-mediated senescence phenotype, we measured the RNA expression levels of several genes belonging to the SASP by qRT–PCR. As expected, the expression of all these genes were upregulated following B-RAF activation, whereas their levels were unaffected or decreased in MIR31HG knockdown cells ( Fig. 3c ). It has been reported previously that p16 INK4A is able to induce cellular senescence without expressing the associated inflammatory phenotype [37] . We therefore speculated whether the cellular senescence observed after MIR31HG depletion was mediated by increased p16 INK4A expression. Indeed, the cell growth phenotype and the formation of SAHFs induced by MIR31HG knockdown could be rescued by p16 INK4A depletion ( Fig. 3d,e and Supplementary Fig. 4a,b ). p16 INK4A activation during senescence results in repression of the transcriptional activity of the E2F transcription factors and, in consequence, of its pro-proliferative target genes. By analysing gene expression by qRT–PCR, we observed that a set of E2F target genes were reduced after MIR31HG depletion to similar levels as in senescence cells ( Supplementary Fig. 4c ), indicating that the cell growth defect observed on MIR31HG knockdown are due to an increased level of p16 INK4A . Moreover, p53 and phosphorylated γH2A.X were not activated by MIR31HG knockdown, indicating the absence of DNA damage ( Supplementary Fig. 4d,e ), which may explain the lack of SASP [36] and supporting a p16 INK4A -dependent senescence phenotype. 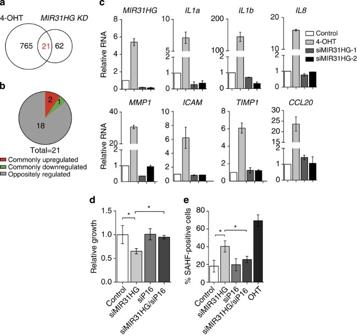Figure 3: The effect ofMIR31HGin senescence is p16INK4Adependent. (a) Venn diagram representing the number of genes altered following 4-OHT treatment and siMIR31HGtransfection after 72 h (log2-fold change >±1.5, false discovery rate (FDR) <0.05). (b) Pie chart showing the number of genes commonly upregulated (red), commonly downregulated (green) or oppositely regulated (grey) by 4-OHT and siRNA knockdown. (c) qRT–PCR analysis of components of the SASP 72 h after 4-OHT treatment or transfection with the siRNAs indicated. (d) Absorbance measurements of crystal violet solution at 560 nM, 72 h post transfection with the indicated siRNAs. (e) Quantification of the number of SAHF-positive cells in cells transfected with the siRNAs or treatment indicated. At least 150 cells from three independent experiments were counted. All the graphs represent the mean±s.e.m. from at least three independent experiments. Student’st-test,*P<0.05,**P<0.01. Figure 3: The effect of MIR31HG in senescence is p16 INK4A dependent. ( a ) Venn diagram representing the number of genes altered following 4-OHT treatment and si MIR31HG transfection after 72 h (log 2 -fold change >±1.5, false discovery rate (FDR) <0.05). ( b ) Pie chart showing the number of genes commonly upregulated (red), commonly downregulated (green) or oppositely regulated (grey) by 4-OHT and siRNA knockdown. ( c ) qRT–PCR analysis of components of the SASP 72 h after 4-OHT treatment or transfection with the siRNAs indicated. ( d ) Absorbance measurements of crystal violet solution at 560 nM, 72 h post transfection with the indicated siRNAs. ( e ) Quantification of the number of SAHF-positive cells in cells transfected with the siRNAs or treatment indicated. At least 150 cells from three independent experiments were counted. All the graphs represent the mean±s.e.m. from at least three independent experiments. Student’s t -test, *P< 0.05, **P< 0.01. Full size image MIR31HG is exported to the cytoplasm during senescence To investigate the mechanisms whereby MIR31HG expression is increased in senescence and how its silencing results in senescence, we performed cellular fractionation in TIG3 cells with and without B-RAF activation. In control cells, MIR31HG was located both in the nucleus and the cytoplasm, with slight enrichment in the nuclear fraction. In contrast, following B-RAF activation, MIR31HG was almost exclusively cytoplasmic ( Fig. 4a ). To bolster these data in an independent cell line, we turned to immortalized primary BJ fibroblasts. As OIS has been shown to be p16 INK4A independent in BJ cells [38] , one hypothesis could be that MIR31HG remains in the nucleus during senescence, thus preventing p16 INK4A expression. To test this hypothesis, we used BJ-hTERT-ER:B-RAF cells, which responded to 4-OHT with an increase of MIR31HG , together with induction of other senescence markers such as IL8 or MMP1 to a similar extent as observed in TIG3 cells ( Supplementary Fig. 5a ). By cellular fractionation, we assessed the distribution of MIR31HG in BJ cells undergoing OIS. Similar to what we observe in TIG3 cells, MIR31HG in BJ cells is located about equally in the nucleus and in the cytoplasm under normal conditions but almost exclusively in the cytoplasm after 72 h 4-OHT-treatment ( Supplementary Fig. 5b ). However, in our hands, these cells also showed an increase of p16 INK4A RNA and protein levels during senescence ( Supplementary Fig. 5c ), in agreement with a relocation of MIR31HG away from the INK4A locus. To further investigate this translocation we carried out cell fractionation assays in a time-course experiment during 4-OHT treatment. We observed that the amount of MIR31HG in control cells remains largely unaltered throughout the treatment period in both compartments ( Fig. 4b ). However, after 36 h of 4-OHT treatment, the levels of nuclear MIR31HG started to decrease ( Fig. 4b , left panel). Inversely, at this time point after the treatment an increase in cytoplasmic MIR31HG was detected ( Fig. 4b , right panel). In the same conditions we measured GAPDH and MALAT1 as cytoplasmic and nuclear controls, respectively, and observed that both transcripts behaved as expected throughout the experiment, with no changes detected in response to 4-OHT treatment ( Supplementary Fig. 5d,e ). 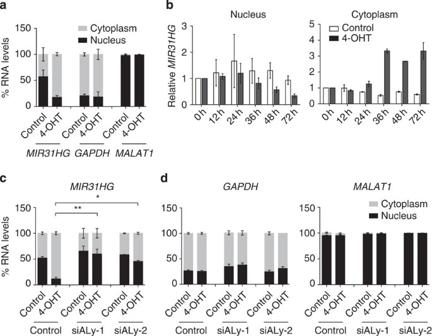Figure 4:MIR31HGis exported to the cytoplasm on senescence induction by a general RNA export pathway. (a) Percentage of nuclear and cytoplasmic RNA levels ofMIR31HG,GAPDHandMALAT1measured by qRT–PCR after subcellular fractionation in cells treated with ethanol (control) or 4-OHT for 72 h. (b) Nuclear (left) and cytoplasmic (right) RNA fraction from total RNA in control cells (white) and 4-OHT-treated cells (black) for the indicated time points. Values at time 0 for both conditions were set as 1. (c) Percentage of nuclear and cytoplasmic RNA levels ofMIR31HGin control or 4-OHT treated cells 72 h after transfection with the indicated siRNAs. (d) Percentage of nuclear and cytoplasmic RNA levels ofGAPDHandMALAT1in the experiment indicated inc. All the graphs show the mean±s.e.m. from at least three independent experiments. Student’st-test,*P<0.05,**P<0.01. Figure 4: MIR31HG is exported to the cytoplasm on senescence induction by a general RNA export pathway. ( a ) Percentage of nuclear and cytoplasmic RNA levels of MIR31HG , GAPDH and MALAT1 measured by qRT–PCR after subcellular fractionation in cells treated with ethanol (control) or 4-OHT for 72 h. ( b ) Nuclear (left) and cytoplasmic (right) RNA fraction from total RNA in control cells (white) and 4-OHT-treated cells (black) for the indicated time points. Values at time 0 for both conditions were set as 1. ( c ) Percentage of nuclear and cytoplasmic RNA levels of MIR31HG in control or 4-OHT treated cells 72 h after transfection with the indicated siRNAs. ( d ) Percentage of nuclear and cytoplasmic RNA levels of GAPDH and MALAT1 in the experiment indicated in c . All the graphs show the mean±s.e.m. from at least three independent experiments. Student’s t -test, *P< 0.05, **P< 0.01. Full size image It has been recently reported that a subset of lncRNAs are exported to the cytoplasm via common mRNA pathways [39] . To corroborate the export of MIR31HG during senescence, we depleted a set of export factors that have been previously involved in RNA export [40] , [41] ( Supplementary Fig. 5f ). Among the factors tested, the knockdown of Aly using two independent siRNAs significantly increased the retention of MIR31HG in the nucleus under senescence induction, indicating that this export factor is involved in MIR31HG export to the cytoplasm ( Fig. 4c,d and Supplementary Fig. 5f–h ). These experiments show that MIR31HG is exported to the cytoplasm in senescence by an Aly-dependent RNA export pathway. MIR31HG is required for PcG binding to the INK4A locus To investigate the role of MIR31HG in regulating p16 INK4A expression, we measured p16 INK4A expression levels from total RNA in the time-course experiment mentioned above. We observed MIR31HG total expression increased up to threefold after 24 h 4-OHT treatment ( Fig. 5a , left panel). However, upregulation of p16 INK4A occurs later ( Fig. 5a , right panel), concomitantly with the decrease in nuclear MIR31HG levels ( Fig. 5b ). 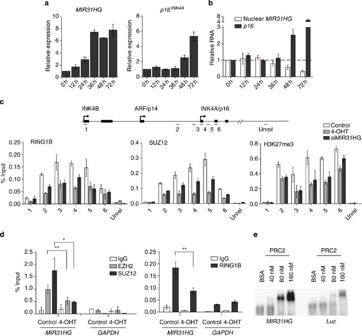Figure 5:MIR31HGis required for PcG binding to theINK4Alocus and interacts with PcG proteins. (a)MIR31HG(left) andp16INK4A(right) RNA levels from total RNA extracted from cells treated with 4-OHT for the time indicated measured by qRT–PCR. The data are represented as the expression in 4-OHT versus control, setting untreated as 1. (b) NuclearMIR31HGlevels from experiment inFig. 4band totalp16INK4Atranscript levels in cells treated with 4-OHT for the indicated time points. The graph represents the data from the treatment versus the control. Levels in cells without treatment have been set to1 (dotted red line). (c) ChIP–qPCR experiments for RING1B, SUZ12 and H3K27me3 throughout theINK4/ARFlocus or at an unrelated region (unrel) in ethanol (control), 4-OHT-treated and siMIR31HG-transfected cells. The position of primers used in the analysis are shown in the schematic diagram (red) and the sequences are present inSupplementary Table 4. (d) RNA immunoprecipitation analysis monitoring EZH2 and SUZ12 (left), and RING1B (right) binding toMIR31HGRNA andGAPDHRNA in control and 4-OHT-treated cells. All the graphs (a–d) show the mean±s.e.m. from three independent experiments. Student’st-test,*P<0.05, **P<0.01. (e) Electrophoretic mobility assay showing thein vitrobinding of 2 nMMIR31HGandLuciferase(Luc) transcript to the indicated amounts of recombinant PRC2 complex. BSA at the highest concentration (160 nM) was used as a negative control. Figure 5: MIR31HG is required for PcG binding to the INK4A locus and interacts with PcG proteins. ( a ) MIR31HG (left) and p16 INK4A (right) RNA levels from total RNA extracted from cells treated with 4-OHT for the time indicated measured by qRT–PCR. The data are represented as the expression in 4-OHT versus control, setting untreated as 1. ( b ) Nuclear MIR31HG levels from experiment in Fig. 4b and total p16 INK4A transcript levels in cells treated with 4-OHT for the indicated time points. The graph represents the data from the treatment versus the control. Levels in cells without treatment have been set to1 (dotted red line). ( c ) ChIP–qPCR experiments for RING1B, SUZ12 and H3K27me3 throughout the INK4/ARF locus or at an unrelated region (unrel) in ethanol (control), 4-OHT-treated and siMIR31HG-transfected cells. The position of primers used in the analysis are shown in the schematic diagram (red) and the sequences are present in Supplementary Table 4 . ( d ) RNA immunoprecipitation analysis monitoring EZH2 and SUZ12 (left), and RING1B (right) binding to MIR31HG RNA and GAPDH RNA in control and 4-OHT-treated cells. All the graphs ( a – d ) show the mean±s.e.m. from three independent experiments. Student’s t -test, *P< 0.05, ** P< 0.01. ( e ) Electrophoretic mobility assay showing the in vitro binding of 2 nM MIR31HG and Luciferase ( Luc ) transcript to the indicated amounts of recombinant PRC2 complex. BSA at the highest concentration (160 nM) was used as a negative control. Full size image Therefore, we investigated a nuclear function for MIR31HG in regulating p16 INK4A expression in normal cells. As p16 INK4A is tightly regulated at the transcriptional level by PcG complexes [25] , [26] , [27] , we hypothesized that MIR31HG participates in PcG-mediated repression. Towards this, we first investigated whether PcG recruitment to the INK4 locus was affected by MIR31HG knockdown. Using chromatin immunoprecipitation (ChIP) experiments, we assessed the binding of RING1B and SUZ12, components of PRC1 and PRC2, respectively, to several regions of the INK4A locus. As expected, RING1B, SUZ12 and the repressive mark established by PRC2, H3K27me3 were present throughout the locus in control cells and with reduced presence in senescent cells ( Fig. 5c and Supplementary Fig. 6a ). Intriguingly, MIR31HG knockdown cells showed a significant reduction in the presence of PRCs and H3K27me3, comparable to that seen in senescence conditions ( Fig. 5c ), which correlates with the increase in p16 INK4A transcription. As controls, we did not observe any RING1B, SUZ12 and H3K27me3 enrichment at different positions of the MIR31HG promoter ( Supplementary Fig. 6b ), nor at an unrelated region located several megabases away ( Fig. 5c ). The amounts of PcG proteins bound to the INK4B locus were also very low and no significant differences were observed on MIR31HG depletion ( Fig. 5c ). MIR31HG interacts with PcG complexes It is well known that lncRNAs can contribute to the recruitment of PcG complexes to repress gene transcription of target genes, and in some cases this regulation may be dependent on direct lncRNA interaction with PcG proteins such as EZH2, SUZ12 and CBX7 (refs 8 , 42 , 43 ). To investigate binding of MIR31HG to PcG complexes, we carried out RNA immunoprecipitation using antibodies towards SUZ12, EZH2 (PRC2) and RING1B (PRC1). MIR31HG bound all three PcG proteins in control cells, suggesting that this transcript is part of the repressive complexes ( Fig. 5d and Supplementary Fig. 6c ). Importantly, this interaction was decreased in senescence ( Fig. 5d and Supplementary Fig. 6c ), consistent with the activation of p16 INK4A transcription and with the reduced levels of MIR31HG in the nucleus after senescence. Although the PRC2 protein levels are decreased in OIS compared with control cells, we did not observe differences in the amount of protein immunoprecipitated in both conditions ( Supplementary Fig. 6d and data not shown). Next, we investigated whether MIR31HG was able to directly interact with PcGs. Using in-vitro -transcribed full-length MIR31HG and purified recombinant reconstituted PRC2 complex ( Supplementary Fig. 6e ), we performed RNA electrophoretic mobility shift assays. Adding increasing amounts of PRC2 to 2nM 32 P-labelled MIR31HG transcript we observed a shift, indicating direct binding of MIR31HG to PRC2 ( Fig. 5e ). Purified BSA was used as a negative protein control. In-vitro interactions with PRC2 have been shown to occur in a promiscuous manner [44] . Indeed, when we used an in-vitro -transcribed Luciferase transcript, we still observed PRC2 binding; however, the strength of the binding is higher for MIR31HG than for Luciferase ( Fig. 5e and Supplementary Fig. 6f ). These results indicate that MIR31HG is able to interact directly with PRC2. MIR31HG interacts with the INK4A and MIR31HG loci To gain more insight into the regulatory mechanism, we investigated RNA–chromatin interactions using chromatin isolation by RNA purification (ChIRP) [45] , [46] . This technique uses biotinylated antisense oligonucleotides to purify endogenous lncRNAs and their associated chromatin complexes. Using two non-overlapping oligonucleotide pools targeting MIR31HG , we were able to enrich MIR31HG but not the negative control mRNA GAPDH ( Fig. 6a ). Almost undetectable levels of transcripts were recovered using oligonucleotides targeting Luciferase mRNA, demonstrating the specificity of the approach ( Fig. 6a ). RNA purification followed by qPCR revealed interactions between MIR31HG RNA and both p16 INK4A and MIR31HG promoters in control cells. Importantly, these interactions were diminished in senescence ( Fig. 6b,c ) and reduced to background levels at an unrelated region situated several megabases away ( Fig. 6d ). 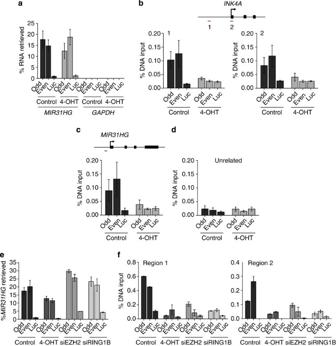Figure 6:MIR31HGinteracts with theINK4AandMIR31HGloci in control cells but not in senescence or in the absence of PcG proteins. (a) ChIRP experiments using two independent probe poolsMIR31HG-asDNA (odd and even) retrieved∼15%–20% ofMIR31HGendogenous RNA and undetectable levels ofGAPDH.Luc-asDNA probes retrieved undetectable levels of both RNAs. ChIRP DNA signal forMIR31HGandLucbinding on theINK4Apromoter (b),MIR31HGpromoter (c) and on an unrelated region (d) in ethanol (control) and 4-OHT-treated cells. Positions of the primers used for qPCR are shown in red and the sequences provided inSupplementary Table 4. All the graphs show the mean±s.e.m. from three independent experiments. (e)MIR31HGretrieval in a ChIRP experiments with the same probes as inbfrom ethanol (control), 4-OHT-treated cells or cells transfected with siRNAs againstEZH2orRING1B. (f) ChIRP DNA signal forMIR31HGbinding at theINK4Apromoter in the conditions described ine. The position of the primers are shown inb. The graphs (e,f) show the mean±s.e.m. from two independent experiments. Figure 6: MIR31HG interacts with the INK4A and MIR31HG loci in control cells but not in senescence or in the absence of PcG proteins. ( a ) ChIRP experiments using two independent probe pools MIR31HG -asDNA (odd and even) retrieved ∼ 15%–20% of MIR31HG endogenous RNA and undetectable levels of GAPDH . Luc- asDNA probes retrieved undetectable levels of both RNAs. ChIRP DNA signal for MIR31HG and Luc binding on the INK4A promoter ( b ), MIR31HG promoter ( c ) and on an unrelated region ( d ) in ethanol (control) and 4-OHT-treated cells. Positions of the primers used for qPCR are shown in red and the sequences provided in Supplementary Table 4 . All the graphs show the mean±s.e.m. from three independent experiments. ( e ) MIR31HG retrieval in a ChIRP experiments with the same probes as in b from ethanol (control), 4-OHT-treated cells or cells transfected with siRNAs against EZH2 or RING1B . ( f ) ChIRP DNA signal for MIR31HG binding at the INK4A promoter in the conditions described in e . The position of the primers are shown in b . The graphs ( e , f ) show the mean±s.e.m. from two independent experiments. Full size image To investigate whether MIR31HG acts together with PRC2 in regulating p16 INKAa expression, we performed ChIRP experiments in RING1b or EZH2 knockdown cells ( Supplementary Fig. 7a ). In these conditions, we could retrieve ∼ 15%–25% of the endogenous transcript ( Fig. 6e ) and observed that MIR31HG interaction with p16 INK4 A promoter is diminished in the absence of PcG ( Fig. 6f ) correlating with p16 INK4A expression ( Supplementary Fig. 7b ). These experiments suggest that MIR31HG and PcG proteins cooperate in repressing INK4A expression. An OIS-activated enhancer interacts with MIR31HG promoter As the above results suggested a possible role for MIR31HG in mediating chromatin looping between MIR31HG and INK4A chromatin regions, situated 400 kb apart, we performed circular chromosome conformation capture followed by deep sequencing (4C-seq) [47] , using the MIR31HG and INK4A promoters as viewpoints. No obvious interaction between these two regions was detected. However, we identified a strong interaction between the MIR31HG promoter and a region located ∼ 100 kb upstream MIR31HG ( Fig. 7a and Supplementary Fig. 8a ). To validate these data, we repeated the 4C-seq experiments using the identified region as a viewpoint and confirmed the existence of a physical interaction between MIR31HG promoter and that chromosomal location ( Fig. 7b and Supplementary Fig. 8a ). Examining ENCODE data, we observed that the identified interacting region contains features characterizing enhancers, such as high levels of the histone marks H3K27ac and H3K4me1, and low presence of H3K4me3. It is also characterized by DNA hypersensitivity and by high transcription factor occupancy (Encode project consortium [48] ( Supplementary Fig. 8b ). To validate the enhancer features in senescent TIG3 cells, we carried out ChIP experiments for H3K4me1 and H3K4me3 in control and senescence cells, respectively. Using seven pairs of primers spanning the 20-kb region, we observed low signals for H3K4me3 and high signals for H3K4me1, as expected for an enhancer, in both situations ( Supplementary Fig. 8c ). However, the levels of H3K4me1 were significantly higher under senescence conditions, suggesting an activation of the enhancer during senescence ( Fig. 7c ). In contrast, in three different regions of the INK4A promoter, H3K4me1 and H3K4me3 levels were similar in control cells and only the levels of H3K4me3 increased in senescence, correlating with the transcriptional activation of p16 INK4A after B-RAF activation ( Fig. 7c ). Recent studies have reported that many enhancers can bidirectionally transcribe non-coding RNAs with low expression levels (enhancer RNAs (eRNAs)) [49] and our RNA-seq data indicated that bidirectional transcription was occurring from the enhancer. By qRT–PCR, we were able to detect these transcripts almost exclusively during senescence ( Fig. 7d ). To corroborate the functionality of these enhancer, we created luciferase reporter constructs carrying different fragments of the 20-kb region, corresponding to peaks in enhancer marks in fibroblast data from ENCODE ( Supplementary Fig. 8b ). As enhancers are shown to act in both directions, we cloned both the forward and the reverse sequences and measured the activation of a luciferase gene driven by the SV40 promoter. A pGL3-basic vector containing both the SV40 promoter and enhancer was used as a positive control. Following transient transfections into TIG3 cells, we observed enhancer activity from the reporters containing fragment 2 and fragment 3 in both directions, but not fragment 1 ( Fig. 7e ). Taken together, these results characterize a new functional enhancer with direct interaction with MIR31HG during senescence. 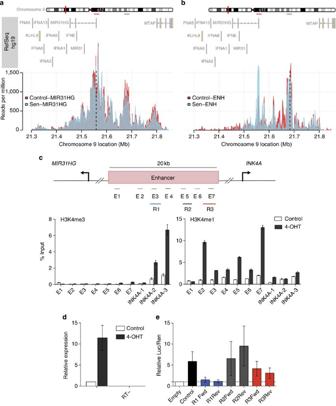Figure 7: A 20-kb enhancer region activated during OIS interacts with theMIR31HGpromoter. (a,b) 4C-seq representation of the chromosome interactions detected usingMIR31HG(a) or the enhancer region (b) as viewpoints. At the top, the ideogram represents the human chromosome 9. The location of the 4C-seq profiles is shown by the vertical red mark. Position ofMIR31HGpromoter is shown in red and the enhancer region in green. RefSeqhg19genes are indicated by rectangles (exons) and arrows (introns) that point the direction of transcription. Interactions occurring in ethanol-treated cells (control) are shown in red and in 4-OHT-treated cells in blue. (c) ChIP–qPCR experiments monitoring H3K4me3 (left) and H3K4me1 (right) binding throughout the enhancer region in ethanol-treated cells (control) (white) and in 4-OHT-treated cells (black). Primer positions are indicated in the diagram and inSupplementary Fig. 8b, and the sequences are provided inSupplementary Table 4. (d) qRT–PCR analysis of an eRNA transcribed from the enhancer identified, in control cells or in 4-OHT-treated cells. The data show the enrichment in senescence compared with control cells. No product was detected when the reverse transcriptase enzyme was omitted. (e) Activation ofLuciferasereporter constructs containing three different fragments of the enhancer cloned in forward (Fwd) and reverse (Rev) orientation. A control plasmid containing SV40 enhancer was used as positive control. Luciferase values normalized toRenilla luciferaseare shown relative to the pGL3-promoter empty vector set as 1 (dotted black line). All the graphs (c–e) show the mean±s.e.m. from at least three independent experiments. Figure 7: A 20-kb enhancer region activated during OIS interacts with the MIR31HG promoter. ( a , b ) 4C-seq representation of the chromosome interactions detected using MIR31HG ( a ) or the enhancer region ( b ) as viewpoints. At the top, the ideogram represents the human chromosome 9. The location of the 4C-seq profiles is shown by the vertical red mark. Position of MIR31HG promoter is shown in red and the enhancer region in green. RefSeq hg19 genes are indicated by rectangles (exons) and arrows (introns) that point the direction of transcription. Interactions occurring in ethanol-treated cells (control) are shown in red and in 4-OHT-treated cells in blue. ( c ) ChIP–qPCR experiments monitoring H3K4me3 (left) and H3K4me1 (right) binding throughout the enhancer region in ethanol-treated cells (control) (white) and in 4-OHT-treated cells (black). Primer positions are indicated in the diagram and in Supplementary Fig. 8b , and the sequences are provided in Supplementary Table 4 . ( d ) qRT–PCR analysis of an eRNA transcribed from the enhancer identified, in control cells or in 4-OHT-treated cells. The data show the enrichment in senescence compared with control cells. No product was detected when the reverse transcriptase enzyme was omitted. ( e ) Activation of Luciferase reporter constructs containing three different fragments of the enhancer cloned in forward (Fwd) and reverse (Rev) orientation. A control plasmid containing SV40 enhancer was used as positive control. Luciferase values normalized to Renilla luciferase are shown relative to the pGL3-promoter empty vector set as 1 (dotted black line). All the graphs ( c – e ) show the mean±s.e.m. from at least three independent experiments. Full size image MIR31HG and p16 INK4A inversely correlate in melanoma MIR31HG has been previously reported to be deregulated in human cancers [34] , [50] , [51] . In our model system, MIR31HG is driven by B-RAF oncogene activation. We therefore hypothesized a role for MIR31HG -mediated p16 INKa regulation in melanoma, where 40%–60% of the patients carry B-RAF mutations. We analysed RNA expression data sets in melanoma tumour samples from The Cancer Genome Atlas (TCGA Research Network: http://cancergenome.nih.gov/ ). In this data set, INK4A is mutated or homozygously deleted in ∼ 40% of cases. The deletions are strongly centred at INK4A , often extending up or downstream of INK4A ; however, MIR31HG is rarely affected. Importantly, focusing exclusively on tumours holding normal diploid INK4A loci with no mutations or copy number changes, we observed a negative correlation between MIR31HG and p16 INK4A RNA expression (Pearson’s r =−0.33, P =0.03, two-tailed test) ( Supplementary Fig. 8d ). This finding suggests that MIR31HG might be repressing p16 INK4A expression in human melanoma. Over the last few years, a number of lncRNAs have been identified and characterized as important factors in fundamental physiological and pathological processes. Here we contribute to the understanding of the function of lncRNAs by describing a role for MIR31HG , which is located 400 kb upstream from the INK4A locus on chromosome 9, in OIS. Consistent with a recent report [50] , MIR31HG downregulation reduces cell growth and, intriguingly, promotes a strong senescence phenotype. Although this may seem paradoxical given the global upregulation of MIR31HG during senescence, our data demonstrates a relative nuclear depletion of MIR31HG during senescence. Here we describe a nuclear function for MIR31HG in repressing the cell cycle inhibitor p16 INK4A at the transcriptional level by facilitating the binding of PcG proteins to the locus. We furthermore show that the general RNA export factor Aly plays a role in the exporting MIR31HG to the cytoplasm during senescence. We do not see changes in Aly RNA or protein levels in senescence. As it has been shown that Aly is methylated to reduce its RNA-binding affinity favouring the downstream export of RNAs [52] , we speculate that Aly is posttranslationally modified during senescence to facilitate MIR31HG export. However, the detailed mechanism by which Aly performs this function requires further investigation. The overexpression of MIR31HG in control cells, where p16 INK4A is already repressed, does not show any evident senescence phenotype. The lack of phenotype, even when the cytoplasmic MIR31HG fraction is increased up to fourfold, suggests that cytoplasmic MIR31HG might not contribute to senescence. We have not been able to revert OIS by overexpressing MIR31HG , although p16 INK4A levels appear to be decreased. This indicates that the mere p16 INK4A reduction in this system is not enough to revert B:RAF-induced senescence. However, MIR31HG knockdown-dependent senescence is reverted by the overexpression, where p16 INK4A is restored to control levels. These results suggest that that p16 INK4A is the main factor in MIR31HG -dependent senescence, while the molecular mechanisms involved in B-RAF-induced senescence might be more complex [53] . As mentioned above, the role of MIR31HG in senescence is dependent on p16 INK4A , as we are able to revert these effects by depleting p16 INK4A . Indeed, the senescence phenotype induced by loss of MIR31HG resembles the p16 INK4A -dependent senescence previously described by the Campisi lab, marked by the absence of both DNA damage and SASP [37] . The MIR31HG regulatory mechanism appears specific for p16 INK4A and not for the other tumour suppressor proteins p15 INK4B and p14 ARF encoded by the INK4-ARF locus. However, we cannot exclude that MIR31HG might be acting in trans affecting other loci. It is currently unclear whether the interaction of MIR31HG with the INK4A locus is direct or mediated by additional factors, such as PcG proteins. Although the MIR31HG transcript contains repetitive sequence elements that might be important for RNA:DNA interactions, as has been shown for Alu elements [54] , [55] , we do not observe any obvious complementarity between MIR31HG and the INK4A locus. Although the MIR31HG transcript binds the genomic regions MIR31HG and INK4A , we could not detect a direct interaction between the two loci using 4C-seq, which in turn rules out a chromatin looping model, as has recently been shown for other lncRNAs [56] , [57] . In contrast, our 4C-seq, as well as previously published HiC-seq data [58] , indicates that the two genes belong to separate topological domains and therefore are likely to not have physiological relevant interactions. Moreover, we do not observe any major changes in chromosome conformation after MIR31HG knockdown, indicating that MIR31HG is not likely to affect the overall chromatin structure of the locus. Hence, the MIR31HG interaction with its own genomic locus might merely reflect nascent transcription. Importantly, our 4C analyses identified chromatin interactions between MIR31HG and different neighbouring regions. The most intriguing interaction corresponds to an enhancer located ∼ 100 kb from MIR31HG , which appears to be functional under normal conditions and further activated during senescence. The interaction appears to already exist in normal cells, allowing a basal MIR31HG expression level. The activation of the enhancer drives MIR31HG upregulation and the increased interaction frequency might play a more humble additive role. The region encompassing the identified enhancer was recently characterized as a putative super enhancer [59] . Enhancers and super enhancers, large clusters of enhancers, have been demonstrated to bind master transcription factors and to interact with genes that define cell identity [59] . Several enhancers have been shown to respond to diverse stimuli such as neuronal depolarization [49] or ERα signalling [60] . In a recent report Rosenfeld and colleagues [61] demonstrated that ERα-responsive enhancers are characterized by the recruitment of a complex of transcription factors. The expression of key transcription factors in response to B-RAF activation may be involved in the enhancer activation. In the functionality assay, we have not observed differences in the activity of the enhancer fragments in proliferating and in senescent cells. This could be due to the massive overexpression of the reporters, a very artificial system. To support our hypothesis that the identified enhancer is active during senescence, we detect transcription from the enhancer primarily during senescence. A large portion of enhancers can be transcribed into eRNAs [49] , which have been proposed to participate in gene activation [9] , [60] , [62] , [63] . Future experiments will address whether these eRNAs play a functional role in the activation of the enhancer and MIR31HG . Enhancers and super enhancers have been described to be responsible for cell identity [59] . An interesting possibility may be that the enhancers activated in specific tissues or specific conditions might be regulating the expression of other lncRNAs that could exert their actions at a genome level, adding a layer of regulation on transcriptional regulation. By analysing melanoma cancer data, we observed that patients with higher levels of MIR31HG often have reduced p16 INK4A expression. In concordance with our results, this suggests that MIR31HG repression of p16 INK4A in these patients favours cancer development. These data and previous reports from other groups link MIR31HG to cancer. In lung and breast cancers MIR31HG was shown to be upregulated [50] , [51] , whereas in triple-negative breast cancer it appears to be downregulated due to promoter hypermethylation [34] . The mechanism for MIR31HG upregulation in breast and lung cancer remains unknown. Analysis of the enhancer status and the correlation between MIR31HG and p16 INK4A in other types of cancer might reveal a general role for MIR31HG in cancer. The implication of MIR31HG in senescence raises the interesting possibility of its involvement in development, although this may be unlikely, as no evidence of p16 INK4A expression has been detected in developmental senescence in mouse embryos [17] . Altogether, our results provide a new mechanism for p16 INK4A transcriptional regulation by the lncRNA MIR31HG . The importance of p16 INK4A as a tumour suppressor emphasizes the relevance of adding new knowledge to the complex regulatory mechanism of the INK4A locus regulation. The identification of new lncRNAs influencing cell cycle regulators or other tumour suppressors will aid to advance our understanding of the basic biology of cancer. Cell cultures, treatments and siRNA transfections The human diploid cell lines TIG3 and BJ were immortalized with telomerase (hTERT) and transduced with a retrovirus generated from pMSCV-ER:B-RAF previously described [35] . Cells were maintained in DMEM medium (Invitrogen) supplemented with 10% fetal bovine serum (Hyclone) and penicillin/streptomycin (Invitrogen). Senescence was induced by treatment with 1 μM 4-OHT (Sigma) 24 h after seeded for at least 48 h (unless otherwise indicated). When additional incubation time was required, media with fresh 4-OHT was added. Control cells were treated with ethanol for the same period of time. siRNA oligonucleotides were transfected at a final concentration of 50 nM by reverse transfection using RNAiMAX (Invitrogen), according to the manufacturer’s instructions. The siRNAs sequences are listed in Supplementary Table 4 . MIR31HG -overexpressing cell lines To generate lentiviral constructs we cloned the full-length MIR31HG sequence into the inducible vector pLVX-TetOne Puro Vector (Clontech). We use In-Fusion HD Cloning designing primers according to the manufacturer’s indications (see primer sequences in Supplementary Table 4 ). For the lentiviral production, HEK293T cells were transfected using Lipofectamine 2000 (Life Technologies) with 7 μg of pLTVX-MIR31HG or pLTVX-empty, together with 6 μg of VsVg and 5 μg Pax8 viral plasmids. After 48 h, supernatants containing the viral particles were filtered through a 0.45-μm filter. Confluent TIG3 cells were then infected with one-third of the viral supernatant and 8 μg μl −1 polybrene. Twenty-four hours post infection, the cells were selected with 1 μg μl −1 puromycin. Cells were maintained in tetracycline-free tested serum (Clontech). For the expression of the lncRNA 100 ng ml −1 doxycicline was used for 72 h, unless otherwise indicated. Luciferase reporter assays For the enhancer reporter assays, three different fragments from the enhancer region were amplified by PCR from genomic DNA (see primer list). The PCR constructs were cloned into the pGL3-promoter Firefly luciferase reporter vector (Promega), using XhoI restriction enzyme (primer sequences are shown in 5). TIG3 cells (3 × 10 5 ) were seeded in a 24-well plate. After 24 h, the cells were transfected using Lipofectamine 3000 (Life Technologies) with 500 ng of the PGL3-promoter, PGL-3 control or the enhancer-luc constructs, together with 150 ng of pRL-Tk Renilla luciferase reporter vector for transfection control and luciferase assay normalization. Six hours after transfection, fresh media containing 1 μM 4-OHT or EtOh as vehicle was added to the cells. Forty-eight hours after treatment Firefly and Renilla luciferase units were measured, using Dual-Glo Luciferase Assay System and GLo-Max Multi Detection System (Promega). Crystal violet staining Cells were seeded and reverse transfected in 12-well plates (NUNC). Twenty-four, 48, 72 and 96 h after transfection, cells were washed twice in PBS and fixed with 10% formalin for 10 min, and stained with 0.1% crystal violet solution. Excess crystal violet stain was removed by several washes with water. The plates were allowed to dry and crystal violet was extracted by the addition of 10% acetic acid. The amount of crystal violet staining was quantified by measurement of the absorbance at 570 nm. Senescence associated β-galactosidase staining Cells were seeded and transfected in 12-well plates (NUNC). After 72 h post transfection, they were fixed and stained using the β-galactosidase staining kit (Cell Signaling), according to the manufacturer’s protocol. EdU incorporation assays and flow cytometry analysis Cells grown in six-well plates (NUNC) were pulsed with EdU (33 uM) for 30 min before fixation. The EdU was detected using Click-IT EdU Alexa Fluor-647 Flow Cytometry Assay Kit (Molecular Probes, Life Technologies), according to the manufacturer’s protocol. Data were generated by flow cytometric analysis of 10,000 cells per treatment. For propidium iodide staining, harvested cells were fixed in 70% ethanol overnight before incubation in propidium iodide and RNase-A solution for 30 min. Data analysis was performed using the FlowJo software (Tree Star, Inc., Ashland, OR, USA). Immunofluorescence Cells were seeded on rounded coverslips placed in 24-well plates (NUNC). Seventy-two hours post transfection, the cells were washed with PBS × 1, fixed in 4% paraformaldehyde (Sigma) for 10 min and then 0.1% Triton X-100 in PBS (Sigma) was added for 10 min. The coverslips were washed twice with PBS × 1, blocked for 30 min with 5% normal goat serum in PBS before incubation with the primary antibodies in 2% normal goat serum for at least 1 h at room temperature. After intensive washing with PBS × 1, the secondary antibody was incubated in 2% goat serum for 1 h at room temperature in the dark. Next, the coverslips were washed, drained and mounted on glass slides using Prolong Gold Antifade Reagent with DAPI (Life Technologies). Antibodies and dilutions are listed in Supplementary Table 5 . Western blot analysis Cells were seeded, reverse transfected in six-well plates (NUNC) and treated the following day with 1 μM 4-OHT or equivalent volumes of ethanol. After 48/72 h, cells were harvested, washed once with PBS and the pellets lysed in RIPA buffer (150 nM NaCl, 0.1% sodium deoxycholate, 0.1% SDS, 50 mm Tris–HCl (pH 8), 1 mM EDTA) containing protease inhibitors (Complete Mini Protease Inhibitor Cocktail; Roche Applied Science). Proteins were separated by electrophoresis in 4%–12% NuPAGE Bis–Tris gels (Invitrogen) and transferred to nitrocellulose membranes. The antibodies used for western blotting are listed in Supplementary Table 5 . Cell fractionation Cells were grown in 15 cm dishes (NUNC). Nuclear/cytoplasmic fractionation was performed using Nuclei EZ Lysis Buffer (Sigma), following the manufacturer’s protocol. RNA extraction and qRT–PCR analysis Total RNA was isolated using Trizol reagent (Invitrogen), treated with TURBO DNase (Ambion, Life Technologies) and reverse transcribed using TaqMan Reverse Transcription kit (Applied Biosystems) with random hexamer primers. Quantitative real-time PCRs were performed using Syber Green PCR Fast PCR Master Mix 2x (Applied Biosystems). The housekeeping genes GAPDH and RPLP0 were used for normalization of qRT–PCR data, unless otherwise stated. For miR-31 qPCR, total RNA was prepared using Trizol reagent and qPCR analysis was performed using TaqMan miRNA assays (Applied Biosystems), using primers for hsa-miR-31 and RNU44 . To calculate the number of molecules per cell, MIR31HG was in vitro transcribed (see in vitro RNA transcription). The concentration of the transcript was measured by A260 values and converted to the number of copies using the molecular weight of the RNA. Dilutions of this transcript were retro-transcribed as described above and the complementary DNA was used as standard curve for qPCR. The primers used for qPCR are listed in Supplementary Table 4 . RNA sequencing TIG3-hTERT-ER:B-RAF were treated with 1 μM 4-OHT or equal volumes of EtOH for 48 h, or they were transfected with Allstar negative control (Qiagen) or MIR31HG siRNAs for 72 h. RNA was extracted from three biological replicates, the quality assessed on the 2100 expert Bioanalyzer (Agilent) and sent for library preparation and sequencing on the Illumina Hiseq2000 by BGI Genomics (Hong Kong). ChIP experiments Cells were fixed with 1% formaldehyde for 10 min. Cross-linking was arrested by adding glycine (0.125 M) for 5 min at room temperature. The cells were subsequently harvested in SDS lysis buffer (0.5% SDS, 100 mM NaCl, 50 mM Tris-Cl pH 8.1, 5 mM EDTA pH 8.0, protease inhibitor mixture Complete (Roche) and 1 mM phenylmethylsulfonyl fluoride (PMSF). Nuclei were pelleted and resuspended in IP buffer (2 volumes SDS lysis buffer:1 volume Triton-X buffer (100 mM Tris-Cl, pH 8.6, 100 mM NaCl, 5 mM EDTA pH 8.0, 5% Triton X-100)). The lysates were sonicated using BIORUPTOR sonicator for 12 cycles of 30 s and centrifuged at maximum speed. The sheared chromatin was diluted to 1 ml with IP buffer and precleared with salmon sperm DNA/recombinant protein A-agarose (Thermo Scientific) for 2 h. One per cent of the sample was used as the input control and the remaining precleared chromatin was incubated overnight with 10 μg by incubation with salmon sperm DNA/protein-A agarose (50% slurry) and centrifugation. The bead pellets were washed in low- or high-salt conditions (0.1% SDS, 1% Triton X-100, 2 mM EDTA pH 8.0, 20 mM Tris-HCl pH 8.0, and 150 mM (low)/500 mM (high) NaCl). The beads were then washed once with LiCl buffer (0.25 M LiCl, 1% NP-40, 1% Na-deoxycholate, 1 mM EDTA and 10 mM Tris-HCl pH 8.0) followed by two washes with Tris-EDTA buffer. Elution buffer (0.1% SDS, 0.1 M NaHCO 3 ) was added to the samples and the cross-linking was reverted by incubation at 68 °C overnight. Samples were incubated 1 h at 37 °C with RNAse A (Sigma) and 45 min at 50 °C with proteinase K (Ambion, Life Technologies). The DNA was purified using Minelute PCR Purification Kit (Qiagen) and then amplified by qPCR using primers listed in Supplementary Table 4 . Native RNA immunoprecipitation Cells were collected in cold PBS by scraping and lysed in lysis buffer (20 mM Tris-HCl pH 7, 150 mM NaCl, 100 mM KCl, 5 mM MgCl 2 , 0.5% Nonidet P-40, SuperaseIn (Ambion, Life Technologies) 100 U ml −1 , dithiothreitol (DTT) 1 mM and 1 × protease inhibitor mixture Complete (Roche)). After centrifugation, NT2 buffer (50 mM Tris pH 7.4, 150 mM NaCl, 1 mM MgCl 2 , 0.05 Nonidet P-40, 200 U ml −1 SuperaseIn (Ambion, Life Technologies), 1 mM DTT, 15 mM EDTA pH 8) was added to the supernatant to 1 ml total volume and the samples were precleared with yeast RNA/recombinant protein A or G-agarose (Thermo Scientific) for 2 h. One per cent of the sample was used as the input control and the remaining extracts were incubated with the corresponding antibodies ( Supplementary Table 5 ) overnight at 4 °C. RNA–antibody complexes were collected by incubation with protein-A or protein-G agarose. After extensive washing, 1/5 of the sample was used for western blotting control and the remaining for RNA extraction and qRT–PCR analysis. In-vitro RNA transcription and labelling Templates containing the T7 promoter were generated by PCR with high-fidelity DNA polymerase (Phusion HF, Thermo Scientific) and the primers listed in Supplementary Table 4 . PCR products were purified from agarose gels and 1 μg of template was in vitro transcribed using T7 RNA polymerase and the MAXIscript kit (Ambion, Life Technologies) for 2 h at 37 °C. After 30 min DNAse treatment with TURBO DNA free at 37 °C, the reactions were stopped by adding 0.5 mM EDTA. Samples were mixed with formamide loading buffer and boiled 3 min at 37 °C before running on 1% agarose gel in 1 × TBE. The RNA products were purified using NucleoSpin Gel and PCR Clean-up kit (Macherey-Nagel) with NTC buffer for RNA extraction. RNAs were dephosphorylated with 1 U of Calf Intestine Alkaline Phosphatase (Invitrogen) and 5′-end labelled with T4 Polynucleotide Kinase (NEB) and γ- 32 P (Perkin Elmer). Labelled RNAs were precipitated following phenol:chloroform extraction. Radiolabelled RNAs were checked on agarose gel in 1 × TBE buffer and quantified. In-vitro binding and electrophoretic mobility assays Final concentration (2 nM) of radiolabelled RNA was adjusted to 5 μl with Milli-Q water, incubated 1 min at 95 °C and cooled on ice for 2 min. RNA was allow to fold for 30 min at 37 °C in binding buffer (50 mM Tris-HCl pH 7.5, 100 mM KCl, 5 mM MgCl2, 0.1 mM CaCl2, 1 mM DTT, 0.1 mg ml −1 BSA, 0.2 mg ml −1 fragmented yeast RNA (Sigma), 5% glycerol, 0.025% bromophenol blue and 0.025% xylene cyanol). The protein was added at the concentrations indicated and the binding reaction was carried out at 30 °C for 30 min. Samples were loaded on a non-denaturing 0.7% agarose gel in cold 1 × TBE buffer. After 90 min at 90 V of gel electrophoresis, the gels were vacuum dried for 90 min at 80 °C and exposed to an Amersham Hyperfilm ECL film. A five-member PRC2 complex was obtained through co-expression of human Ezh2, His+Flag-tagged Eed, Suz12, Aebp2 and Rbbp4 in High Five cells using a baculovirus expression system (pVL1392-derived transfer vector and Sapphire baculovirus DNA (Allele Biotechnology)). The complex was purified on anti-Flag M2 beads (Sigma) ( Supplementary Fig 5e ). Purified BSA (NEB) was used as negative control. Chromatin isolation by RNA purification CHIRP assays were performed as previously described [46] . Probe design . The antisense oligonucleotide probes were designed using the online probe designer at single molecule fish ( www.singlemoleculefish.com ) using the following parameters: (1) number of probes: 1/100 bp of RNA length; (2) target GC%=45; (3) oligonucleotide length=20; (4) spacing length=60–80. The probes, modified at 3′-end with BiotinTEG were obtained from Stanford University ( http://pan.stanford.edu ). To assess the specificity of the oligonucleotides, the probes were divided into two pools, odd and even. All the experiments were carried out using both pools independently. Antisense oligonucleotides targeting luciferase RNA were used as negative control. RNA immunoprecipitation . Cells (15 × 10 7 ) were grown in 15 cm dishes (NUNC), harvested by trypsinization and cross-linked using 1% glutaraldehyde for 15 min. The cross-linking was quenched by the addition of 1.25 M glycine at room temperature for 5 min. The cells were lysed with 1 ml per 100 mg cell pellet of lysis buffer (50 mM Tris-HCl pH 7, 10 mM EDTA, 1% SDS, 1 mM PMSF, 200 U ml −1 SuperaseIn (Ambion, Life Technologies) and 1 × protease inhibitor mixture Complete (Roche)) and sonicated using BIORUPTOR sonicator for 75 cycles of 30 s. Sonicated samples were centrifuged at 16100, r.c.f. for 10 min and 1% of the lysate was removed as RNA input and DNA input. Two millilitres of hybridization buffer (750 mM NaCl, 1% SDS, 5 mM Tris-HCl pH 7, 1 mM EDTA, 15% formamide, 1 mM PMSF, 200 U ml −1 SuperaseIn (Ambion, Life Technologies) and 1 × protease inhibitor mixture Complete (Roche)) together with 100 pmol of each pool of probes were added to 1 ml of chromatin, mixed and incubated at 37 °C for 4 h, while shaking. RNA was pulled down using the DynaMag-2 magnet strip after incubating with C1 magnetic beads (Invitrogen, Life Technologies) for 30 min at 37 °C, while rotating. Pre-warmed washing buffer (2 × NaCl and sodium citrate, 0.5% SDS and 1 mM PMSF) was used to wash the beads. After the last wash, 100 μl were used for RNA isolation and 900 μl for DNA fraction. RNA isolation . RNA samples were treated with Proteinase K (Ambion, Life Technologies) in PK Buffer (100 mM NaCl, 10 mM Tris-HCl pH 7.0, 1 mM EDTA and 0.5% SDS) at 50 °C for 45 min while shaking and then boiled for 10 min at 95 °C, and RNA was extracted using TRIzol and MIRNeasy mini columns (Qiagen), and then treated with DNase (Qiagen). One microlitre of RNA was used for qRT–PCR analysis, to confirm RNA retrieval. Glyceraldehyde 3-phosphate dehydrogenase (GAPDH) is used as a negative control. DNA isolation . DNA was eluted with Elution Buffer supplemented with RNase A (10 mg ml −1 ) and 10 μl RNase H (10 U μl −1 ) per ml of DNA Elution Buffer (50 mM NaHCO 3 and 10% SDS). After PK treatment at 50 °C for 45 min, DNA was isolated using PhOH:Chloroform:Isoamyl (Sigma) and used for subsequent qPCR analysis with primers indicated in Supplementary Table 4 . 4C and high-throughput sequencing The 4C-seq protocol was followed essentially as previously described [64] . Briefly, 10 7 cells were cross-linked with 4% formaldehyde in PBS/10% FBS for 10 min at room temperature. After quenching the reaction with 0.125 M glycine, cells were lysed in lysis buffer (50 mM Tris pH 7.5, 150 mM NaCl, 5 mM EDTA, 0.5% Igepal, 1%Triton X-100, 1 mM PMSF and protease inhibitor mixture Complete (Roche)) using a douncer. The cross-linked DNA was digested with a 4-bp cutter restriction enzyme site ( Dpn II and Nla III) followed by proximity ligation and cross-linking removal. A secondary restriction enzyme digestion was performed with a 4-bp restriction enzyme ( Nla III and Csp 6l, respectively) followed again by proximity ligation. Primers from the 4C-seq primer database [47] with additional 5′ overhangs of the adapter sequences for Illumina single-read sequencing were used as viewpoint. The sequences are listed in Supplementary Table 4 . Sixteen PCR reactions were carried out using 200 ng of the resulting 4C template per reaction. The products were pooled together and purified using QIAquick PCR purification kit (Qiagen). The quality was assessed using a 2100 expert Bioanalyzer (Agilent) and the samples were sent for deep sequencing using Illumina HiSeq2000 by BGI Genomics (Hong Kong). Bioinformatic analysis For the RNA-seq analysis, we ran TopHat (ref1) (v. 2.0.10) in single-end mode with the option library-type=fr-secondstrand. No GTF file was given to Tophat. Bowtie [65] (v. 2.1.0.0) and SAMtools [66] (v. 0.1.19.0) were called by TopHat. For the differential expression analysis, we used the pipeline [67] . Briefly, bam file output from TopHat were sorted and converted to SAM files using SAMtools and reads per gene were counted using HTSeq with a GTF file from GENCODE [68] (v. 15), with all pseudogenes removed. EdgeR [69] was used for differential expression analysis. Genes with less than one read per million in more than three samples were removed before analysis. Pairwise contrasts were calculated between all experimental groups (see RNA sequencing). For analysis of MIR31HG and p16 INK4 A expression levels in human melanoma tumours, we used molecular profiles of 226 melanoma tumour samples from The Cancer Genome Atlas. We used DNA copy number calls and somatic mutations from the cbioportal (PMID 22588877) to exclude samples with altered INK4A copy number or with mutations targeting INK4A . These filters selected 43 INK4A wild-type tumour samples for further mRNA expression analysis ( Supplementary Table 3 ). We used normalized RNA-seq read counts estimated by the RSEM algorithm (21816040; http://gdac.broadinstitute.org/runs/analyses__2013_09_23/data/SKCM/20130923/ ). We then estimated expression levels of individual genes by computing using log2 read counts per million from the RSEM-normalized read counts in each sample. The 4C-seq mapping and normalization was carried out as described in van de Werken et al. [47] In brief, the 4C-Seq reading primer sequences were demultiplexed from the 4C-seq data and trimmed, from the 5′-end to the first restriction enzyme recognition site. The sequences were mapped, while ignoring quality score, to a database of digested genome fragment ends using the human reference genome build hg19. The interactions near the viewpoint were used to calculate the mean of the normalized coverage for a running window of size 5 kb (indicated by a black line) and a sliding window of 2–50 kb (colour coded in multiscale domainogram [70] . All mean values represent enrichment compared with the maximum 5-kb mean value The 20th and 80th percentiles were computed and depicted in grey areas around the 5-kb running window ( Supplementary Fig. 7a ). The 4C-seq contact profile comparison plots ( Fig. 7a,b ) were generated by combining the mapping [64] and normalization [47] as described previously. A running trimmed mean of 10% was calculated to smoothen the 4C-seq data. The R statistical package version 3.1.0 was used for the statistical calculations and for generating the 4C-seq plots. (R-Core-Team: R: A language and environment for statistical computing. Vienna, Austria: R Foundation for Statistical Computing; 2013). The R Gviz package version 1.8.4. was used for plotting the annotation data. Accession codes : The data associated with the manuscript have been deposited with the accession number: SRP051359 . How to cite this article: Montes, M. et al. The lncRNA MIR31HG regulates p16 INK4A expression to modulate senescence. Nat. Commun. 6:6967 doi: 10.1038/ncomms7967 (2015).